NR2F1 controls tumour cell dormancy via SOX9- and RARβ-driven quiescence programmes Metastases can originate from disseminated tumour cells (DTCs), which may be dormant for years before reactivation. Here we find that the orphan nuclear receptor NR2F1 is epigenetically upregulated in experimental head and neck squamous cell carcinoma (HNSCC) dormancy models and in DTCs from prostate cancer patients carrying dormant disease for 7–18 years. NR2F1-dependent dormancy is recapitulated by a co-treatment with the DNA-demethylating agent 5-Aza-C and retinoic acid across various cancer types. NR2F1-induced quiescence is dependent on SOX9, RARβ and CDK inhibitors. Intriguingly, NR2F1 induces global chromatin repression and the pluripotency gene NANOG, which contributes to dormancy of DTCs in the bone marrow. When NR2F1 is blocked in vivo , growth arrest or survival of dormant DTCs is interrupted in different organs. We conclude that NR2F1 is a critical node in dormancy induction and maintenance by integrating epigenetic programmes of quiescence and survival in DTCs. A large proportion of patients diagnosed with cancer harbour nonproliferative residual tumour cells, which can fuel incurable local or distant recurrences [1] . The ability of dormant residual tumour cells to persist but also interconvert between dormancy and proliferation may be the result of epigenetic reprogramming mechanisms [2] . However, mechanisms and markers that identify dormant cells at risk of resuming growth are unavailable. We reported that p38α/β regulates a quiescence transcription factor (TF) network that contains proliferation/growth arrest and pluripotency/self-renewal genes [3] , [4] , [5] . The p38α/β pathway and quiescence were activated by TGFβ2 signalling specifically in disseminated tumour cells (DTCs) that are dormant in the bone marrow [6] . Further, the p38α/β-regulated TF network served as a ‘dormancy signature’ that was enriched in oestrogen receptor (ER)-positive luminal over ER-negative basal-type primary breast tumours [7] and predicted for longer metastasis-free periods in the ER+ group [7] . Thus, we hypothesized that genes within this signature may influence the timing of metastasis via regulation of dormancy. Among the genes in the dormancy signature [3] , [6] , [7] we identified NR2F1 , an orphan nuclear receptor [8] that induces cell lineage determination in response to signals like retinoic acid (RA) [9] , limits induced pluripotent stem cells (iPS) reprogramming [4] and regulates enhancer elements during human neural crest cell differentiation [10] . Because these processes regulate pluripotency and limit proliferation, we investigated whether NR2F1 and these processes were linked to the interconversion between cancer cell dormancy and proliferation. Like other genes in the RA pathway (for example, RARβ) [11] NR2F1 mRNA is downregulated in several cancers including HNSCC, prostate, lung and breast versus normal tissues (Oncomine database) [12] , [13] , [14] , [15] , [16] and it is functionally linked to a breast cancer susceptibility locus (Mcs1) [17] . Further, upregulation of NR2F1 correlated with longer disease-free periods after hormonal ablation in prostate cancer [18] . Thus, changes in NR2F1 levels in primary tumours may influence residual tumour cell fate. Here we provide evidence that NR2F1 coordinates gene expression found in quiescent cells and also in self-renewing ES cells [19] . We show that NR2F1 regulates the behaviour of residual tumour cells in postoperative mice as its inactivation causes a rapid switch from dormancy to proliferation of occult tumour cells and systemic recurrence. This is true except in the bone marrow, where NR2F1 appears to regulate DTC survival. Importantly, restoration of NR2F1 expression using DNA-demethylating agents and activation of RA signalling is sufficient to recapitulate the quiescence programme and induce chromatin changes linked to a durable dormant state. These findings break new ground in our understanding of the dormancy mechanisms and identify markers that might pinpoint residual cancer with the ability to escape dormancy. NR2F1 high human tumour cells are dormant We first used the squamous cell carcinoma cell line HEp3 model of proliferation versus dormancy to dissect the molecular mechanisms of conversion of malignant cells into a dormancy-like behaviour characterized by tumour cell quiescence [3] , [6] , [20] , [21] , [22] , [23] , [24] , [25] . Proliferating (T-HEp3) cells obtained from tumours and kept in culture reprogramme into a dormant/quiescent phenotype (D-HEp3 cells) after prolonged passaging in vitro . However, this dormant phenotype is not manifested in vitro but it is observed only after injection of D-HEp3 cells in vivo in nude mice s.c. or in the chicken embryo chorioallantoic membrane (CAM). In these in vivo settings the dormant phenotype of D-HEp3 cells can persist for months before reactivation [3] , [6] , [20] , [26] . We compared the expression profiles of deeply quiescent D-HEp3 cells that form small nodules that do not change in size in vivo or proliferative T-HEp3 cells that form growing tumour masses in vivo [3] , [20] and found that NR2F1 was induced approximately threefold in the former cells ( Fig. 1a —see also methods for access to full expression profiles). This was corroborated by immunohistochemistry (IHC), immunofluorescence (IF; Fig. 1b , Supplementary Fig. 1a ) and western blot (WB), where nuclear NR2F1 protein was three- to fourfolds higher in D-HEp3 cells than in T-HEp3 cells ( Fig. 1b ). This was also true for other genes in the RA pathway (RARβ) [27] ( Fig. 1a , Supplementary Fig. 1b ). In two additional aggressive HNSCC cell lines, FaDu and SQ20B [28] , NR2F1 protein and mRNA levels were barely detectable ( Fig. 1b ). Thus, NR2F1 is downregulated in T-HEp3, FaDu and SQ20B HNSCC cells in vitro and tumours in vivo (T-HEp3) when compared with dormant D-HEp3 cells in vitro and dormant nodules in vivo . 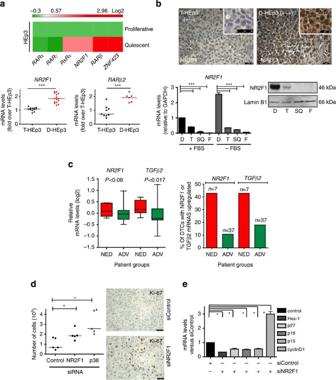Figure 1:  NR2F1 and RA responsive genes in quiescent HEp3 cells. (a) Upper panel: RNA from sorted GFP-positive T-HEp3 (proliferative) and D-HEp3 (quiescent) cells grown in CAMs for 7 days was expression profiled using the Affymetrix platform. The heat map shows the Log2-fold mRNA level change normalized to the levels in proliferative HEp3 cells. Tumours (n=5) were collected and RNA pooled and run in triplicate Affymetrix HG-U133-PLUS2 arrays. Lower panel: QPCR for NR2F1 (T-HEp3 tumoursn=12, D-HEp3 tumoursn=15) and RARβ2 (T-HEp3 tumoursn=9, D-HEp3 tumoursn=6) mRNA in T- and D-HEp3 cells grown in CAMs for 7 day. (b) IHC for NR2F1. Upper panels, T-HEp3 tumours and D-HEp3 nodules sectioned and stained by IHC against NR2F1. Insets, higher magnification of replicate T- or D-HEp3 tumours. Scale bars, 50 μm. Lower left panel: QPCR for NR2F1 mRNA in D, D-HEp3; F, FaDu; SQ, SQ20B; T, T-HEp3 cells in the presence or absence of 10% FBS.n=3 RNA replicates per condition. Lower right panel: nuclear fraction lysates of the indicated cell lines IB for NR2F1. LaminB1, loading control. Three independent experiments. Scale bars, 50 μm. (c) Single-cell expression profiling on bone marrow DTCs. Left panel: BM DTCS were isolated from patients with NED (n=4 patients) and patient with ADV (n=6 patients). Single-cell gene expressions were analysed by Agilent 4 × 44 K Human Microarrays, and NR2F1 and TGFβ2 mRNA levels were compared between both groups. Right panel: percentage of DTCs with high levels of NR2F1 mRNA levels were plotted for NED patients or ADV patients.n=number of DTCs.Pvalues were obtained by Mann–Whitney test. (d) NR2F1 function in D-HEp3 cell dormancy. Left panel: Control, NR2F1- or p38α-depleted D-HEp3 cells were inoculated into CAMs, and 4 days later the total tumour cells were counted. Right panel: IHC for Ki67 in siControl or siNR2F1 tumour sections.n=5 tumours per group. (e) QPCR for HES-1, p27, p16, p15 and cyclinD1 genes from siControl or siNR2F1 tumour RNA samples. Unless stated, all data are representative of at least triplicate independent experiments±s.d.,n=3 RNA replicates per condition unpairedt-test, *P<0.05, ***P<0.0005. Mann–Whitney test was used forin vivoexperiments. Figure 1:  NR2F1 and RA responsive genes in quiescent HEp3 cells. ( a ) Upper panel: RNA from sorted GFP-positive T-HEp3 (proliferative) and D-HEp3 (quiescent) cells grown in CAMs for 7 days was expression profiled using the Affymetrix platform. The heat map shows the Log 2 -fold mRNA level change normalized to the levels in proliferative HEp3 cells. Tumours ( n =5) were collected and RNA pooled and run in triplicate Affymetrix HG-U133-PLUS2 arrays. Lower panel: QPCR for NR2F1 (T-HEp3 tumours n =12, D-HEp3 tumours n =15) and RARβ2 (T-HEp3 tumours n =9, D-HEp3 tumours n =6) mRNA in T- and D-HEp3 cells grown in CAMs for 7 day. ( b ) IHC for NR2F1. Upper panels, T-HEp3 tumours and D-HEp3 nodules sectioned and stained by IHC against NR2F1. Insets, higher magnification of replicate T- or D-HEp3 tumours. Scale bars, 50 μm. Lower left panel: QPCR for NR2F1 mRNA in D, D-HEp3; F, FaDu; SQ, SQ20B; T, T-HEp3 cells in the presence or absence of 10% FBS. n =3 RNA replicates per condition. Lower right panel: nuclear fraction lysates of the indicated cell lines IB for NR2F1. LaminB1, loading control. Three independent experiments. Scale bars, 50 μm. ( c ) Single-cell expression profiling on bone marrow DTCs. Left panel: BM DTCS were isolated from patients with NED ( n =4 patients) and patient with ADV ( n =6 patients). Single-cell gene expressions were analysed by Agilent 4 × 44 K Human Microarrays, and NR2F1 and TGFβ2 mRNA levels were compared between both groups. Right panel: percentage of DTCs with high levels of NR2F1 mRNA levels were plotted for NED patients or ADV patients. n =number of DTCs. P values were obtained by Mann–Whitney test. ( d ) NR2F1 function in D-HEp3 cell dormancy. Left panel: Control, NR2F1- or p38α-depleted D-HEp3 cells were inoculated into CAMs, and 4 days later the total tumour cells were counted. Right panel: IHC for Ki67 in siControl or siNR2F1 tumour sections. n =5 tumours per group. ( e ) QPCR for HES-1, p27, p16, p15 and cyclinD1 genes from siControl or siNR2F1 tumour RNA samples. Unless stated, all data are representative of at least triplicate independent experiments±s.d., n =3 RNA replicates per condition unpaired t -test, * P <0.05, *** P <0.0005. Mann–Whitney test was used for in vivo experiments. Full size image To determine the function of NR2F1 in quiescent D-HEp3 cells in vivo [3] , we performed NR2F1 knockdown via short interfering RNA (siRNA) and found that NR2F1 promoted D-HEp3 cell exit from dormancy and tumour growth, comparable to a siRNA to p38α, as shown for other TFs in the p38α/β-regulated network [3] , [6] ( Fig. 1d , Supplementary Fig. 1c ); no differences were observed in potency of phenotype between siNR2F1 and sip38α. Exit from dormancy coincided with downregulation of cell cycle inhibitors such as p16, p27, p15 and HES-1, all genes involved in quiescence [29] , [30] ( Fig. 1e ). Further, NR2F1 depletion also induced upregulation of cyclinD1 levels and Ki67 staining indicative of G0 exit. To test the potential human implications of these findings, we next tested whether NR2F1 was re-expressed in prostate cancer DTCs [31] . We chose prostate cancer because this cancer type is known to undergo prolonged dormancy phases and because NR2F1 is commonly downregulated in prostate primary tumours [15] , [16] , but may become upregulated after hormonal ablation, which is thought to lead to residual disease dormancy [18] . To this end, we compared individual prostate cancer DTCs isolated via EpCAM marking from the bone marrow of post-radical prostatectomy patients with no evidence of disease (NED—dormant disease) or advanced proliferative disease (ADV). NED patients showed undetectable PSA level (<0.1 ng ml −1 ) 7–18 years after prostatectomy. ADV patients showed disease progression with failed treatment or existing distant metastasis. Seven EpCAM+ individual NED cells (four patients) and 37 ADV cells (six patients) were processed for expression profiling as indicated in Supplementary Table I and Experimental Procedures [31] . When comparing NED versus ADV PCa DTCs we found that 42.8% of NED DTCs showed NR2F1 upregulation versus 10.3% in ADV patient-derived DTCs ( Fig. 1c ). The average mRNA levels for NR2F1 showed a trend towards upregulation ( P <0.08) in NED versus the ADV patient-derived DTCs ( Fig. 1c ). A significant difference in mRNA levels ( P <0.0117) was found for TGFβ2 (ref. 6 ) another dormancy gene we recently linked to bone marrow (BM) DTC dormancy that was also more frequently upregulated in NED versus ADV DTCs (42.8% NED versus 18% ADV; Fig. 1c ). We conclude that dormancy genes found upregulated in HNSCC experimental models (this study and ref. 6 ) are also found upregulated in DTCs from PCa patients carrying dormant disease. Epigenetic regulation of NR2F1 expression IHC analysis showed that compared with benign adjacent oral mucosa NR2F1 expression was absent or low in primary ( n =15) or recurrent ( n =9) HNSCC tumours ( Fig. 2a and Supplementary Fig. 1d,e ) and patient-matched lymph node metastases ( n =11; Fig. 2a ). Further, while 27% of squamous cells in benign adjacent tissues were NR2F1 high (7–66% range), only 1.5±2.5% of tumour cells in primary and recurrent lesions were NR2F1 high . These results show that overall NR2F1 is downregulated in tumour tissues and the intratumour heterogeneity of expression is very low ( Fig. 2a and Supplementary Fig. 1d,e ). Primary tumour tissues showed that 67% of the tumour cells were Ki67+ and none expressed NR2F1, suggesting that proliferative tumour cells are negative for NR2F1 ( Supplementary Fig. 1e ). The overall downregulation of NR2F1 in tumour versus normal squamous tissues is in accord with the expression profiling study [12] where NR2F1 was downregulated in ~85% ( n =41) of HNSCC primary tumours and in ~86% ( n =16) local recurrences. NR2F1 mRNA and protein levels were also lower in human breast carcinoma tissues and in the breast tissue of 20-week-old MMTV-Neu and -Myc mice ( Supplementary Fig. 2a–c ), which at this age develop pre-malignant atypical ductal hyperplasia (ADH) and ductal carcinoma in situ (DCIS)-like lesions [32] . Further, in at least three studies [13] , [33] , [34] including the breast cancer TCGA showed that in ~80% tumour samples NR2F1 was significantly downregulated versus normal tissue (for example, P <1.06 × 10 −25 —TGCA data as measured using a t -Test—Oncomine source). 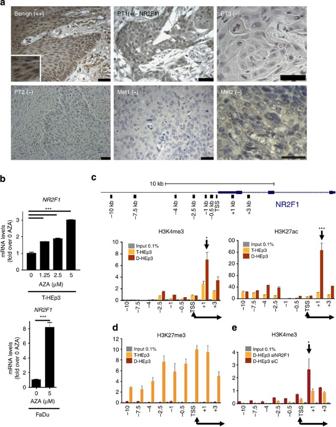Figure 2: NR2F1 expression in HNSCC tumours and epigenetic regulation. (a) NR2F1 protein detection in benign adjacent oral mucosa (inset, magnification of NR2F1+ epithelium), in primary tumours (PT) and lymph node metastasis (met). Scale bars, 50 μm. Images shown are representative ofn=6 benign adjacent tissue, 15 primary tumours, 9 recurrences and 11 metastasis. (b) Azacytidine treatment and NR2F1 expression in HNSCC cells. T-HEp3 (top panel) and FaDu (lower panel) cells were treated with 5-azadeoxycytidine (AZA) at the indicated concentrations for 2 days, and NR2F1 mRNA quantified by QPCR.yaxis, AZA conditions over no AZA. ***P<0.0005, unpairedt-test.n=3 RNA samples per condition. (c,d) H3PTMs at the NR2F1 locus in T- and D-HEp3 cells. T- and D-HEp3 cells were culturedin vitrofollowed by ChIP–qPCR analysis of the NR2F1 genomic locus for H3K4me3, H3K27ac (c) and H3K27me3 (d) histone modifications. Top scheme shows the primers used around the TSS of the NR2F1 genomic locus. Bar graphs indicate fold enrichment over input (1%), *P<0.05, **P<0.005, unpairedt-test, mean±s.d. (n=3). Arrows show sites with significant changes for the indicated histone modification in two independent experiments. All other data are representative of at least triplicate independent experiments. (e) ChIP–qPCR for H3k4me3 at the NR2F1 locus in D-HEp3 cells. After NR2F1 ablation (by siRNA, 50 nM) cultured cells were subjected to ChIP–qPCR for H3K4me3 at the NR2F1 locus. Arrows show sites with significant changes for the indicated histone modification in two independent experiments. *P<0.05, unpairedt-test, mean±s.d. (n=3). All other data are representative of at least triplicate independent experiments±s.d. Figure 2: NR2F1 expression in HNSCC tumours and epigenetic regulation. ( a ) NR2F1 protein detection in benign adjacent oral mucosa (inset, magnification of NR2F1+ epithelium), in primary tumours (PT) and lymph node metastasis (met). Scale bars, 50 μm. Images shown are representative of n =6 benign adjacent tissue, 15 primary tumours, 9 recurrences and 11 metastasis. ( b ) Azacytidine treatment and NR2F1 expression in HNSCC cells. T-HEp3 (top panel) and FaDu (lower panel) cells were treated with 5-azadeoxycytidine (AZA) at the indicated concentrations for 2 days, and NR2F1 mRNA quantified by QPCR. y axis, AZA conditions over no AZA. *** P <0.0005, unpaired t -test. n =3 RNA samples per condition. ( c , d ) H3PTMs at the NR2F1 locus in T- and D-HEp3 cells. T- and D-HEp3 cells were cultured in vitro followed by ChIP–qPCR analysis of the NR2F1 genomic locus for H3K4me3, H3K27ac ( c ) and H3K27me3 ( d ) histone modifications. Top scheme shows the primers used around the TSS of the NR2F1 genomic locus. Bar graphs indicate fold enrichment over input (1%), * P <0.05, ** P <0.005, unpaired t -test, mean±s.d. ( n =3). Arrows show sites with significant changes for the indicated histone modification in two independent experiments. All other data are representative of at least triplicate independent experiments. ( e ) ChIP–qPCR for H3k4me3 at the NR2F1 locus in D-HEp3 cells. After NR2F1 ablation (by siRNA, 50 nM) cultured cells were subjected to ChIP–qPCR for H3K4me3 at the NR2F1 locus. Arrows show sites with significant changes for the indicated histone modification in two independent experiments. * P <0.05, unpaired t -test, mean±s.d. ( n =3). All other data are representative of at least triplicate independent experiments±s.d. Full size image We next tested whether NR2F1 might be downregulated by DNA promoter methylation. Treatment of T-HEp3 and FaDu cells that express negligible levels of NR2F1 with 5-azadeoxycytidine (5-Aza-C), strongly increased NR2F1 mRNA expression by more than threefold without any toxicity ( Fig. 2b and Supplementary Fig. 2d ). However, analysis of DNA promoter methylation showed no differences in CpG island methylation between T-HEp3 and D-HEp3 cells ( Supplementary Fig. 2e ). Chromatin immunoprecipitation (ChIP) analysis covering a region spanning −10 to +3 Kb of the transcription start site (TSS) of the NR2F1 gene revealed that the H3K4me3 and H3K27ac transcriptional activation marks are highly enriched at the NR2F1 TSS in D-HEp3 as compared with T-HEp3 cells ( Fig. 2c ). In contrast, the H3K27me3 repressive mark was enriched in the promoter of NR2F1 in T-HEp3 cells ( Fig. 2c ). These changes in H3-PTMs correlated with the NR2F1 mRNA levels in T- versus D-HEp3 HNSCC cells. ChIP analysis for the same H3-PTMs mentioned above in D-HEp3 cells with and without NR2F1 knockdown showed that on its own promoter at least H3K4me3 seems to be regulated by NR2F1 (+1 position; Fig. 2d ). We conclude that DNA promoter methylation in regions not covered by our analysis and/or changes in histone-H3-PTMs and transcriptional activation contribute to NR2F1 silencing in proliferative T-HEp3 cells. NR2F1 regulates SOX9 and RARβ during dormancy TF network analysis of gene profiles regulated by p38α/β [3] identified 40 co-regulated genes with predicted or validated binding elements for NR2F1 in their promoters ( Supplementary Fig. 3a , Supplementary Table II ). Ten of these genes contained both NR2F1 and RARβ (a target of NR2F1 (ref. 35 )) binding sites. These genes were upregulated >2.8-fold in D-HEp3 cells both in culture and in vivo ( Fig. 3a and Fig. 1a ). We focused on SOX9 because its promoter is bound by NR2F1 and RARβ [10] and it is a RA- and p38α/β-responsive TF [3] , [36] , linked to growth inhibition and differentiation [37] . Accordingly, overexpression in T-HEp3 cells with an active MKK6 mutant (p38 activator), upregulated SOX9, NR2F1 and RARβ mRNAs ( Supplementary Fig. 3b ). Further, NR2F1 overexpression in T-HEp3 cells greatly increased the activity of a SOX9-luciferase reporter ( Supplementary Fig. 3c ), suggesting that SOX9 is a direct target of NR2F1. Finally, we show that as in Fig. 2c knockdown of NR2F1 reduced the presence of H3K4me3 marks in the promoters of SOX9 and RARβ in dormant D-HEp3 cells ( Supplementary Fig. 3d ) without affecting H3K27me3 marks in any tested promoter (not shown). Thus, NR2F1 is in part responsible for inducing active transcription H3-PTMs in its own promoter and that of its target genes ( Supplementary Fig. 3d ). 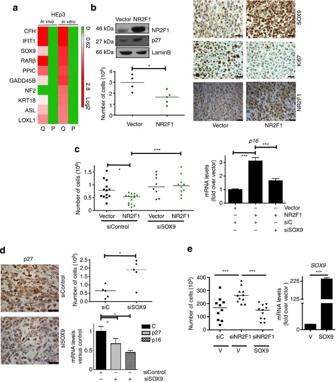Figure 3: Identification of NR2F1 and RARβ targets. (a) Heat map for the 10 genes that share NR2F1 and RARβ-binding elements. Log2 gene expression changes, green, basal expression in Proliferative (P) T-HEp3 cells and increasing red intensity indicates upregulation in quiescent (Q) D-HEp3 cells. (b) Overexpression of NRF21 inhibits tumour growth. NR2F1, p27 and Lamin-B detection in T-HEp3 cells transfected with NR2F1 or Control plasmids (top left panels) or tested for tumour growth on CAMs for 5 days (bottom left panel).n=4 tumours per group. IHC on vector or NR2F1-overexpressing tumour sections for the indicated antigens (right panels). Scale bars, 50 μm. (c) NR2F1 inhibits tumour growth via SOX9. Left panel: T-HEp3 cells transfected with SOX9 or control siRNAs (50 nM) were re-transfected with empty or NR2F1 cDNA vectors. Tumour growth was quantified 4 days later on CAMs; three independent experiments (left panel). Vector,n=13 tumours; siC NR2F1,n=15 tumours; siSOX9 vector,n=8 tumours; siSOX9 NR2F1,n=10 tumours. Right panel: p16 mRNA levels relative to tubulin in T-HEp3 cells in the indicated groups. (d) SOX9 RNAi promotes D-HEp3 cell proliferation. D-HEp3 cells were transfected with siRNA for SOX9 or control (siC, 50 nM). Left: tumour sections from siControl and siSOX9 groups stained for p27 by IHC. Top right: growth of siControl or siSOX9-treated D-HEp3 cells on CAMs for 4 days. Bottom right: mRNA levels for p27 and p16 after 4 daysin vivo.n=5 tumours per group. Scale bars, 50 μm. (e) SOX9 overexpression blocks reactivation from dormancy after NR2F1 RNAi. Left panel: D-HEp3 cells were transfected with NR2F1 or control siRNAs (50 nM) and then transfected with SOX9 cDNA or empty vector. Growth of these groups was assessed on CAMs for 4 days. Two independent experiments. Right panel: D-HEp3 cells were transfected with SOX9 cDNA or empty vector. SOX9 mRNA levels were measured by QPCR. siC vectorn=10 tumours; siNR2F1 vector,n=11 tumours; siNR2F1 SOX9n=11 tumours. Unless stated, all data are representative of at least triplicate independent experiments±s.d.,n=3 RNA replicates per condition unpairedt-test, *P<0.05, ***P<0.0005. Mann–Whitney test was used forin vivoexperiments. Figure 3: Identification of NR2F1 and RARβ targets. ( a ) Heat map for the 10 genes that share NR2F1 and RARβ-binding elements. Log2 gene expression changes, gree n , basal expression in Proliferative (P) T-HEp3 cells and increasing red intensity indicates upregulation in quiescent (Q) D-HEp3 cells. ( b ) Overexpression of NRF21 inhibits tumour growth. NR2F1, p27 and Lamin-B detection in T-HEp3 cells transfected with NR2F1 or Control plasmids (top left panels) or tested for tumour growth on CAMs for 5 days (bottom left panel). n =4 tumours per group. IHC on vector or NR2F1-overexpressing tumour sections for the indicated antigens (right panels). Scale bars, 50 μm. ( c ) NR2F1 inhibits tumour growth via SOX9. Left panel: T-HEp3 cells transfected with SOX9 or control siRNAs (50 nM) were re-transfected with empty or NR2F1 cDNA vectors. Tumour growth was quantified 4 days later on CAMs; three independent experiments (left panel). Vector, n =13 tumours; siC NR2F1, n =15 tumours; siSOX9 vector, n =8 tumours; siSOX9 NR2F1, n =10 tumours. Right panel: p16 mRNA levels relative to tubulin in T-HEp3 cells in the indicated groups. ( d ) SOX9 RNAi promotes D-HEp3 cell proliferation. D-HEp3 cells were transfected with siRNA for SOX9 or control (siC, 50 nM). Left: tumour sections from siControl and siSOX9 groups stained for p27 by IHC. Top right: growth of siControl or siSOX9-treated D-HEp3 cells on CAMs for 4 days. Bottom right: mRNA levels for p27 and p16 after 4 days in vivo . n =5 tumours per group. Scale bars, 50 μm. ( e ) SOX9 overexpression blocks reactivation from dormancy after NR2F1 RNAi. Left panel: D-HEp3 cells were transfected with NR2F1 or control siRNAs (50 nM) and then transfected with SOX9 cDNA or empty vector. Growth of these groups was assessed on CAMs for 4 days. Two independent experiments. Right panel: D-HEp3 cells were transfected with SOX9 cDNA or empty vector. SOX9 mRNA levels were measured by QPCR. siC vector n =10 tumours; siNR2F1 vector, n =11 tumours; siNR2F1 SOX9 n =11 tumours. Unless stated, all data are representative of at least triplicate independent experiments±s.d., n =3 RNA replicates per condition unpaired t -test, * P <0.05, *** P <0.0005. Mann–Whitney test was used for in vivo experiments. Full size image NR2F1 overexpression mimicked dormancy in T-HEp3 cells, as it induced growth suppression, a reduction in Ki67 levels and induction of p27 and SOX9 proteins and p16 and SOX9 mRNAs ( Fig. 3b,c , Supplementary Fig. 3e ). Importantly, SOX9 was required for NR2F1-induced quiescence as RNA interference (RNAi) to SOX9 in T-HEp3 cells completely blocked NR2F1-dependent induction of growth suppression ( Fig. 3c ). This was accompanied by a decrease in p16 levels ( Fig. 3c ). An siRNA against SOX9 in D-HEp3 cells also promoted tumour growth and decreased p16 and p27 mRNA levels and p27 protein levels ( Fig. 3d , Supplementary Fig. 3f ), but no changes were observed in p15 and HES-1 levels (not shown; Fig. 3d ). SOX9 was sufficient to induce dormancy because overexpression of a cDNA encoding human SOX9 completely reversed the pro-proliferative effects of NR2F1 siRNA on D-HEp3 cells ( Fig. 3e ). Since RA regulates NR2F1 expression [38] , we tested whether the pan-RAR ligand atRA, increased NR2F1 and its target genes. We found that RARβ, SOX9 and NR2F1 itself were induced between 1.3- and 4-fold in T-HEp3 and FaDu cells, in response to 48-h treatment with atRA ( Fig. 4a and Supplementary Fig. 4a ). NR2F1 depletion in T-HEp3 cells reduced atRA-induced upregulation of RARβ and SOX9 and even basal levels of SOX9 were further reduced upon NR2F1 and RARβ knockdown ( Supplementary Fig. 4b ). 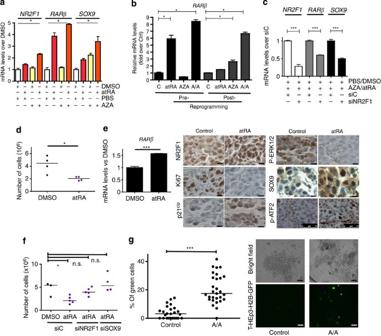Figure 4: AzaC+atRA and NR2F1-induced reprogramming. (a) T-HEp3 cells treated with 5 nM of AzaC or PBS for 48 h in media+charcolized serum were washed and stimulated with atRA (2 μM) or DMSO for 48 h in serum-free media. NR2F1, RARβ and SOX9 mRNA levels were measured by QPCR. *P<0.05. (b) T-HEp3 cells were treated as ina. Then, cells were grown in DMEM, 10% FBS for 3 days without drugs and RARβ mRNA levels measured by QPCR. Pre-reprogramming, 4 days of Aza+atRA treatment (seeSupplementary Fig. 4f); post reprogramming, 3 days after Aza+atRA treatment. *P<0.05. (c) NR2F1, RARβ and SOX9 mRNA levels in T-HEp3 cells transfected with siControl or siNR2F1 (50 nM) treated as inaand left untreated for 3 days. *P<0.05. (d) T-HEp3 cells were stimulated with atRA (2μM) or DMSO inoculated on CAMs (150 × 103per animal), and tumour growth scored on day 4.n=4, *P<0.05. (e) Sections from tumours treated as indwere probed for RARβ mRNA levels or stained for the indicated antigens. ***P<0.0005. Scale bars, 15 and 75 μm. (f) T-HEp3 cells transfected with siRNAs for NR2F1, SOX9 or control were stimulated with atRA (2 μM) or DMSO and then inoculated into CAMs (1.5 × 105cells per embryo) as ind. *P<0.05. siC DMSO group,n=3 tumours; siC atRA group,n=5 tumours; siNR2F1 atRA group,n=5 tumours; siSOX9 atRA group,n=4 tumours. (g) Quantification (left) of H2B-GFP label retaining T-HEp3 cellsin vivoafter treatment as ina,except that 3 days before the treatment cells were induced with doxycycline to induce H2B-GFP; ***P<0.0001. Right: phase contrast (top) and GFP channel (bottom) images of H2B-GFP tumour explants after gentle mechanical mincing. Unless stated, all data are representative of at least triplicate independent experiments.y=percentage of positive green cells in four fields.n=6 tumours per group. Scale bars, 45 μm. Unless stated, all data are representative of at least triplicate independent experiments±s.d.,n=3 RNA replicates per condition unpairedt-test. Mann–Whitney test was used forin vivoexperiments. Figure 4: AzaC+atRA and NR2F1-induced reprogramming. ( a ) T-HEp3 cells treated with 5 nM of AzaC or PBS for 48 h in media+charcolized serum were washed and stimulated with atRA (2 μM) or DMSO for 48 h in serum-free media. NR2F1, RARβ and SOX9 mRNA levels were measured by QPCR. * P <0.05. ( b ) T-HEp3 cells were treated as in a . Then, cells were grown in DMEM, 10% FBS for 3 days without drugs and RARβ mRNA levels measured by QPCR. Pre-reprogramming, 4 days of Aza+atRA treatment (see Supplementary Fig. 4f ); post reprogramming, 3 days after Aza+atRA treatment. * P <0.05. ( c ) NR2F1, RARβ and SOX9 mRNA levels in T-HEp3 cells transfected with siControl or siNR2F1 (50 nM) treated as in a and left untreated for 3 days. * P <0.05. ( d ) T-HEp3 cells were stimulated with atRA (2μM) or DMSO inoculated on CAMs (150 × 10 3 per animal), and tumour growth scored on day 4. n =4, * P <0.05. ( e ) Sections from tumours treated as in d were probed for RARβ mRNA levels or stained for the indicated antigens. *** P <0.0005. Scale bars, 15 and 75 μm. ( f ) T-HEp3 cells transfected with siRNAs for NR2F1, SOX9 or control were stimulated with atRA (2 μM) or DMSO and then inoculated into CAMs (1.5 × 10 5 cells per embryo) as in d . * P <0.05. siC DMSO group, n =3 tumours; siC atRA group, n =5 tumours; siNR2F1 atRA group, n =5 tumours; siSOX9 atRA group, n =4 tumours. ( g ) Quantification (left) of H2B-GFP label retaining T-HEp3 cells in vivo after treatment as in a, except that 3 days before the treatment cells were induced with doxycycline to induce H2B-GFP; *** P <0.0001. Right: phase contrast (top) and GFP channel (bottom) images of H2B-GFP tumour explants after gentle mechanical mincing. Unless stated, all data are representative of at least triplicate independent experiments. y =percentage of positive green cells in four fields. n =6 tumours per group. Scale bars, 45 μm. Unless stated, all data are representative of at least triplicate independent experiments±s.d., n =3 RNA replicates per condition unpaired t -test. Mann–Whitney test was used for in vivo experiments. Full size image We next explored the effect of 5-Aza-C on NR2F1 induction of target genes. Both RARβ and SOX9 induction in T-HEp3 and FaDu cells was strongly enhanced by the treatment ( Supplementary Fig. 4c,d ). Interestingly, NR2F1 overexpression was not sufficient to upregulate RARβ mRNA ( Supplementary Fig. 4e ) but pretreatment with 5-Aza-C followed by NR2F1 overexpression now made the T-HEp3 cells permissive to RARβ upregulation by exogenous NR2F1 above the effect of 5-Aza-C alone ( Supplementary Fig. 4e ). Accordingly, in T-HEp3 cells treated with a combination of low-dose of Aza-C (5 nM) + atRA ( Supplementary Fig. 4f ), NR2F1 , SOX9 and RARβ mRNAs were significantly upregulated ( Fig. 4a ). The effect of atRA on RARβ was transient and its expression returned to pre-induction levels 3 days after atRA washout ( Fig. 4b ). In contrast, when cells were pre-treated with AzaC (5 nM) followed by atRA (2 μM), the induced levels of RARβ were maintained even after atRA removal for 3 days ( Fig. 4b ). The AzaC + atRA treatment was also able to induce RARβ expression across various cancer cell line subtypes ( Supplementary Fig. 5a ). Importantly, the sustained expression of RARβ and SOX9 in these conditions required NR2F1 expression as tested in T-HEp3, MCF-7 and SQ20B cells ( Fig. 4c and Supplementary Fig. 5a ). These results argue that in carcinoma cell lines from different tissues, AzaC-plus-atRA-induced gene expression is durable and dependent on NR2F1. AtRA and 5-Aza-C treatment induces dormancy To expand the above experiments, we queried whether treatment of T-HEp3 cells with atRA would induce the key hallmarks of reprogramming into quiescence in vivo . Treatment with atRA for 5 days resulted in inhibition of tumour growth in vivo using the chicken chorioallantoic membrane assays for rapid in vivo readout [20] ( Fig. 4d ). Growth inhibition was with no apparent change in apoptosis or senescence ( Supplementary Fig. 5b ). Analysis of the tumour tissue from CAMs showed that atRA treatment caused a marked upregulation of dormancy genes. These included upregulation of RARβ and p21 mRNAs and NR2F1 and SOX9 proteins ( Fig. 4e ) and downregulation of Ki67 and P-ERK1/2 levels ( Fig. 4e ), suggesting a G0 arrest. Treatment with atRA also increased the phosphorylation of ATF2, a downstream p38 target ( Fig. 4e ) suggesting a low ERK/p38 activity ratio [20] . Importantly, in T-HEp3 cells RNAi to SOX9 and NR2F1 were sufficient to eliminate the growth inhibitory effect of atRA in vivo ( Fig. 4f ). However, as expected ( Fig. 4b ), atRA-treated T-HEp3 cells that were growth inhibited for 1 week, escaped this inhibition by atRA after a second week in vivo ( Supplementary Fig. 5c ). We next tested whether the persistent effect of combined 5-Aza-C+atRA treatment in culture ( Fig. 4b ) could induce prolonged T-HEp3 quiescence state in vivo . We used a Tet-ON-inducible H2B-GFP-tagged T-HEp3 line where doxycycline (DOX) induces H2B-GFP and upon de-induction and DNA replication only cells that are quiescent are H2B-GFP-positive. H2B-GFP-tagged T-HEp3 cells treated only in vitro with 5-Aza-C+atRA for 4 days were then followed on CAMs for 6 days ( Fig. 4g ). In this sequence the 5-Aza-C+atRA treatment induced a persistent dormant phenotype that lasted for at least 2 weeks in vivo ( Supplementary Fig. 5d ). This correlated with the percentage of H2B-GFP-positive cells in AzaC+atRA-treated cells that was approximately fivefold greater at 6 days than in vehicle-treated cells ( Fig. 4g ). Together, these data argue that restoring NR2F1 , RARβ and SOX9 expression during the AzaC+atRA reprogramming phase could induce a sustained (at least 2 weeks) dormant phenotype. NR2F1 regulates expression of pluripotency genes NR2F1 regulates lineage commitment and differentiation [10] and it was shown to block iPS reprogramming [4] . However, whether NR2F1 affects pluripotency gene expression upon dormancy onset is unknown. We found that both NANOG and SOX2 mRNAs were significantly upregulated in dormant BM-HEp3 (ref. 6 and D-HEp3 cells over the proliferative T-HEp3 and Lu-HEp3 (ref. 6 )) cells ( Fig. 5a ). Furthermore, NANOG and SOX2 mRNAs were strongly induced by the AzaC+atRA treatment and siRNAs to NR2F1 completely eliminated this induction ( Fig. 5b ). The induction of these pluripotency genes by the Aza+atRA reprogramming protocol was not correlated with tumour-initiating capacity as this reprogramming inhibited the ability of T-HEp3 cells to form tumour spheres in stem cell media ( Supplementary Fig. 5e ). NR2F1 also inhibited tumour growth of MMTV-Myc mammary tumour cells, where overexpression of NR2F1 significantly reduced tumorigenicity in mice and tumour sphere formation ( Fig. 5c,d and Supplementary Fig. 6a ). We conclude that induction of pluripotency genes by NR2F1 in dormant cancer cells is associated with a growth-suppressive or quiescent behaviour and not with immediate tumour-initiating capacity. 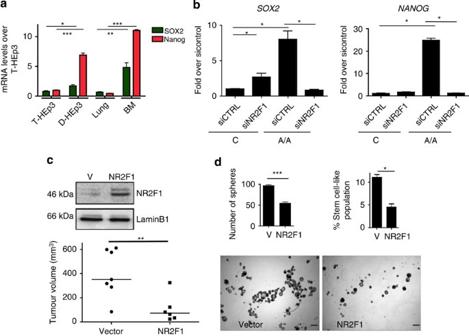Figure 5: NR2F1 and tumour-initiating properties. (a) Expression of SOX2 and NANOG in proliferative versus dormant HEp3 sublines. Cells were grown in complete medium and RNA was extracted and converted to cDNA. SOX2 and NANOG mRNA levels were measured by QPCR. ***P<0.0005, *P<0.05, **P<0.005, unpairedt-test. Lung: a line derived from HEp3 lung DTCs (proliferative). BM: a line derived from HEp3 BM DTCs (dormant). (b) AzaC+atRA treatment requires NR2F1 to induce SOX2 and NANOG. T-HEp3 cells treated with AzaC+atRA or PBS/DMSO were transfected with siControl or siNR2F1, and SOX2 and NANOG mRNAs were detected by QPCR. (c) NR2F1 inhibits MMTV-Myc tumour sphere formation capacity. MMTV-myc cells stably expressing an empty vector control or murine NR2F1 cDNA were inoculated orthotopically in syngeneic FvB mouse (1,000 cells per mouse). Tumour size was measured daily and the final tumour size is shown. In all panels, experiments were performed a minimum of two times. V, vector, *P<0.05, unpairedt-test.N=6 per condition,y=tumour volume. (d) Same cells as in panelc, were cultured in mammosphere conditions and quantified (top left), and 8 days later cells were analysed by FACS for CD29 high and CD24-low markers (top right), and quantified and imaged (bottom left and right). Pictures show MMTV-myc mammoespheres. V, vector, ***P<0.0005, unpairedttest.n=3 wells per condition,y=number of spheres per conditions. Scale bars, 200 μm. Unless stated, all data are representative of at least triplicate independent experiments±s.d. and QPCR:n=3 RNA replicates per condition. Mann–Whitney test was used forin vivoexperiments. Figure 5: NR2F1 and tumour-initiating properties. ( a ) Expression of SOX2 and NANOG in proliferative versus dormant HEp3 sublines. Cells were grown in complete medium and RNA was extracted and converted to cDNA. SOX2 and NANOG mRNA levels were measured by QPCR. *** P <0.0005, * P <0.05, ** P <0.005, unpaired t -test. Lung: a line derived from HEp3 lung DTCs (proliferative). BM: a line derived from HEp3 BM DTCs (dormant). ( b ) AzaC+atRA treatment requires NR2F1 to induce SOX2 and NANOG. T-HEp3 cells treated with AzaC+atRA or PBS/DMSO were transfected with siControl or siNR2F1, and SOX2 and NANOG mRNAs were detected by QPCR. ( c ) NR2F1 inhibits MMTV-Myc tumour sphere formation capacity. MMTV-myc cells stably expressing an empty vector control or murine NR2F1 cDNA were inoculated orthotopically in syngeneic FvB mouse (1,000 cells per mouse). Tumour size was measured daily and the final tumour size is shown. In all panels, experiments were performed a minimum of two times. V, vector, * P <0.05, unpaired t -test. N =6 per condition, y =tumour volume. ( d ) Same cells as in panel c , were cultured in mammosphere conditions and quantified (top left), and 8 days later cells were analysed by FACS for CD29 high and CD24-low markers (top right), and quantified and imaged (bottom left and right). Pictures show MMTV-myc mammoespheres. V, vector, *** P <0.0005, unpaired t test. n =3 wells per condition, y =number of spheres per conditions. Scale bars, 200 μm. Unless stated, all data are representative of at least triplicate independent experiments±s.d. and QPCR: n =3 RNA replicates per condition. Mann–Whitney test was used for in vivo experiments. Full size image NR2F1 high cells display a global repressive chromatin state We showed that tumor-initiating cells display an open chromatin state (H3K27me3 low , H3K9me3 low , H3K4me3 low ), while non-tumour-initiating cells displayed a reverse profile and a more repressive or ‘bivalent’ chromatin state [28] . NR2F1 could regulate local changes in H3-PTMs in its own and SOX9 and RARβ promoters, but the global effect of NR2F1 on chromatin marks was not obvious. IHC and IF analyses showed that in contrast to T-HEp3 cells (NR2F1 low ), D-HEp3 cells (NR2F1 high ) showed a H3K9me3 high and H3K27me3 high profile ( Fig. 6a ). Accordingly, the AzaC+atRA reprogramming protocol rendered T-HEp3 cells H3K27me3 high /H3K9me3 high /H3K4me3 low /NR2F1 high /SOX9 high and quiescent in vivo ( Fig. 6b,c , Supplementary Figs 5d and 6b , Fig. 4g ); this effect was evident up to 8 days after drugs washout when these tumour cells are still nonproliferative. Importantly, basal H3-PTMs (K9me3 and K27me3) levels and the global changes in H3-PTMs induced by the reprogramming were NR2F1-dependent ( Fig. 6d ). 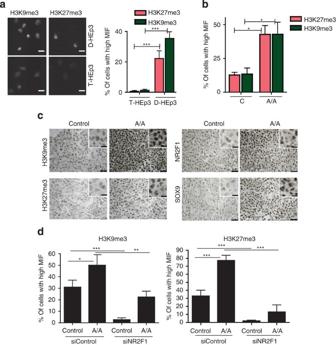Figure 6: NR2F1 and global H3-PTMs. (a) H3K27me3 and H3K9me3 levels in T- and D-HEp3 cells. D-HEp3 and T-HEp3 cells grown on coverslips were fixed with 4% PFA and stained with anti-H3K27me3 and -H3K9me3 antibodies (left panels); representative images are shown. Quantification (right panel) was performed after setting up fixed arbitrary units of immunoflourescence intensity. High mean intensity (MIF) fluorescence was scored using Metamorph for each group. ***P<0.0005, unpairedt-test. Scale bars, 40 μm. (b) Effect of AzaC+atRa treatment on H3K27me3 and H3K9me3 levels. T-HEp3 cells grownin vitrowere treated with AzaC+atRA or PBS/DMSO as described inFig. 4awere stained for the indicated markers and percent of high MFI cells scored. *P<0.05, unpairedt-test. (c) AzaC+atRa treatment renders T-HEp3 cells [H3K27me3/H3K9me3/NR2F1/SOX9]highin vivo. T-HEp3 cells were treated with AzaC+atRa as described inSupplementary Fig. 4f, and 1 day after washout cells were inoculated into CAMs (150 × 103cells per embryo). One week later, tumours were collected and histological sections were stained by IHC using the indicated antibodies. Scale bars, 50 μm. Insets show higher magnification views. Scale bars, 50 μm, insets=15 μm. (d) NR2F1 is required to induce high H3K9me3 and H3K27me3 levels after AzaC+atRa treatment. T-HEp3 cells were transfected with siControl or siNR2F1 and then treated with AzaC+atRA or PBS/DMSO as described inSupplementary Fig. 4f. Three days after reprogramming, cells were fixed and stained for the indicated markers. ***P<0.0005, **P<0.005, *P<0.05, unpairedt-test. Unless stated, all data are representative of at least triplicate independent experiments±s.d. Fora,b,d,n=200 cells,y=percentage of cells with high MIF. Figure 6: NR2F1 and global H3-PTMs. ( a ) H3K27me3 and H3K9me3 levels in T- and D-HEp3 cells. D-HEp3 and T-HEp3 cells grown on coverslips were fixed with 4% PFA and stained with anti-H3K27me3 and -H3K9me3 antibodies (left panels); representative images are shown. Quantification (right panel) was performed after setting up fixed arbitrary units of immunoflourescence intensity. High mean intensity (MIF) fluorescence was scored using Metamorph for each group. *** P <0.0005, unpaired t -test. Scale bars, 40 μm. ( b ) Effect of AzaC+atRa treatment on H3K27me3 and H3K9me3 levels. T-HEp3 cells grown in vitro were treated with AzaC+atRA or PBS/DMSO as described in Fig. 4a were stained for the indicated markers and percent of high MFI cells scored. * P <0.05, unpaired t -test. ( c ) AzaC+atRa treatment renders T-HEp3 cells [H3K27me3/H3K9me3/NR2F1/SOX9] high in vivo . T-HEp3 cells were treated with AzaC+atRa as described in Supplementary Fig. 4f , and 1 day after washout cells were inoculated into CAMs (150 × 10 3 cells per embryo). One week later, tumours were collected and histological sections were stained by IHC using the indicated antibodies. Scale bars, 50 μm. Insets show higher magnification views. Scale bars, 50 μm, insets=15 μm. ( d ) NR2F1 is required to induce high H3K9me3 and H3K27me3 levels after AzaC+atRa treatment. T-HEp3 cells were transfected with siControl or siNR2F1 and then treated with AzaC+atRA or PBS/DMSO as described in Supplementary Fig. 4f . Three days after reprogramming, cells were fixed and stained for the indicated markers. *** P <0.0005, ** P <0.005, * P <0.05, unpaired t -test. Unless stated, all data are representative of at least triplicate independent experiments±s.d. For a , b , d , n =200 cells, y =percentage of cells with high MIF. Full size image NR2F1 regulates residual tumour cell fate post-tumour surgery We next studied whether NR2F1 could dictate DTC fate. After primary tumour surgery, HEp3 cells form overt metastases in lungs and lymph nodes [20] , [39] . In contrast, in the bone marrow and spleen DTCs are detectable, but overt metastases never develop [6] . In addition, at least 2 months after surgery, local recurrences develop in <17% of animals. Inducible knockdown of NR2F1 in Tet-ON-sh-NR2F1-miR-T-HEp3 cells was >60% after DOX treatment ( Supplementary Fig. 6c,d ), without changes in its close related homologue NR2F2 levels ( Supplementary Fig. 6d ). Strikingly, sh-NR2F1-miR induction resulted in vigorous development of local tumour recurrences (33%; n =15), while in mice without DOX treatment recurrences were fewer (17% n =11) and developed later ( Fig. 7a ). After take, sh-NR2F1-miR ‘ON’ tumours also grew much faster than the sh-NR2F1-miR ‘OFF’ controls reaching a much larger volume ( Supplementary Fig. 6e ). We also found that AzaC+atRA-induced tumour growth inhibition was blocked by the activation of the sh-NR2F1-miR in HEp3 cells ( Fig. 7b ). Thus, residual tumour cells may remain dormant and express high levels of NR2F1. Accordingly, residual solitary tumour cells in surgery margins showed upregulation of NR2F1 and SOX9, while the proliferation marker P-H3 was absent ( Fig. 7a ). These data argue that dormant NR2F1 hi / SOX9 hi /P-H3 lo residual solitary tumour cells exist in surgery margins. 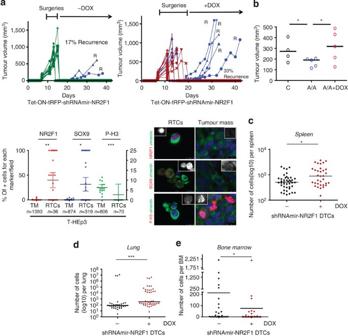Figure 7: Effect of NR2F1 knockdown on locoregional and distant recurrences. (a) Upper panels: Tet-ON-inducible shRNAmir-NR2F1 T-HEp3 s.c. tumours that reached ~800 mm3in nude mice were surgically removed and the mice were treated with (25 mg kg−1DOX, every 48 h,n=15) or without (N=12, middle panel) DOX (right panel). Flat green or red lines on thexaxis are all animals without recurrences. Lower left panel: skin sections in surgery margins (48 h after surgeries) were analysed by IF. T-HEp3 cells were identified by vimentin staining (green). NR2F1, SOX9 and P-H3 (red) were stained with specific antibodies. Graph, % of positive cells for each marker per field. RTC, single residual tumour cell; TM, tumour mass;n=total number of cells counted in two to five animals. The lower right panel shows representative pictures for each antigen. Inset: higher magnification of cells in the red channel (grey scale pseudocolour). TM,n=3 animals, RTCs,n=3 animals; for SOX9: TM,n=3 animals, RTCs,n=5 animals; for P-H3: TM,n=2 animals, RTCs,n=3 animals. Scale bars, 10 μm. (b) NR2F1 knockdown and AzaC+atRA(A/A)-induced dormancy. T-HEp3 cells treatedin vitrowith PBS/DMSO (c, control) or A/A treatment were inoculated into nude mice (n=5) and then treated as ina; 12 days later, tumour growth was measured. *P<0.05, unpairedt-test. (c) Effect of NR2F1 knockdown on spleen DTCs. DTCs isolated from the spleen of the same animals inawere detected by Alu-QPCR as described6Mann–Whitney testP<0.05. SPLEN DTCs:n=14 mice control,n=11 mice shNR2F1,y=Ctvalues in triplicate per mice. (d) Effect of NR2F1 knockdown on lung DTCs. The same animals inawere used to detect DTCs from the lung by Alu-QPCR. Mann–Whitney testP<0.05. Lung DCTS:n=11 mice control,n=14 mice shNR2F1,y=Ctvalues in triplicate per mice. (e) Effect of NR2F1 knockdown on BM DTCs. BM aspirates from same animals inawere used to detect BM DTCs by Alu-QPCR. Mann–Whitney testP<0.05. BM DTCs:n=10 mice control,n=12 mice shNR2F1y=Ctvalues in triplicate per mice. Unless stated, all data are representative of at least duplicate independent experiments±s.d. Figure 7: Effect of NR2F1 knockdown on locoregional and distant recurrences. ( a ) Upper panels: Tet-ON-inducible shRNAmir-NR2F1 T-HEp3 s.c. tumours that reached ~800 mm 3 in nude mice were surgically removed and the mice were treated with (25 mg kg −1 DOX, every 48 h, n =15) or without ( N =12, middle panel) DOX (right panel). Flat green or red lines on the x axis are all animals without recurrences. Lower left panel: skin sections in surgery margins (48 h after surgeries) were analysed by IF. T-HEp3 cells were identified by vimentin staining (green). NR2F1, SOX9 and P-H3 (red) were stained with specific antibodies. Graph, % of positive cells for each marker per field. RTC, single residual tumour cell; TM, tumour mass; n =total number of cells counted in two to five animals. The lower right panel shows representative pictures for each antigen. Inset: higher magnification of cells in the red channel (grey scale pseudocolour). TM, n =3 animals, RTCs, n =3 animals; for SOX9: TM, n =3 animals, RTCs, n =5 animals; for P-H3: TM, n =2 animals, RTCs, n =3 animals. Scale bars, 10 μm. ( b ) NR2F1 knockdown and AzaC+atRA(A/A)-induced dormancy. T-HEp3 cells treated in vitro with PBS/DMSO (c, control) or A/A treatment were inoculated into nude mice ( n =5) and then treated as in a ; 12 days later, tumour growth was measured. * P <0.05, unpaired t -test. ( c ) Effect of NR2F1 knockdown on spleen DTCs. DTCs isolated from the spleen of the same animals in a were detected by Alu-QPCR as described [6] Mann–Whitney test P <0.05. SPLEN DTCs: n =14 mice control, n =11 mice shNR2F1, y = C t values in triplicate per mice. ( d ) Effect of NR2F1 knockdown on lung DTCs. The same animals in a were used to detect DTCs from the lung by Alu-QPCR. Mann–Whitney test P <0.05. Lung DCTS: n =11 mice control, n =14 mice shNR2F1, y = C t values in triplicate per mice. ( e ) Effect of NR2F1 knockdown on BM DTCs. BM aspirates from same animals in a were used to detect BM DTCs by Alu-QPCR. Mann–Whitney test P <0.05. BM DTCs: n =10 mice control, n =12 mice shNR2F1 y = C t values in triplicate per mice. Unless stated, all data are representative of at least duplicate independent experiments±s.d. Full size image Importantly, when we monitored DTC burden after primary tumour surgery using human-specific Alu -sequence qPCR, we found that by reducing NR2F1 levels (upon DOX treatment) we could increase the median number of tumour cells in spleens and lungs by two to fivefold ( Fig. 7c,d ). Because this is performed after primary tumour surgery and there is no more cell dissemination, this result suggests that the observed increase in the number of tumour cells/organ may be because of re-awakening of dormant DTCs after NR2F1 knockdown. The detection of 0.5–6 × 10 6 lung tumour cells is correlated with the presence of metastasis as reported previously at these time points [6] , [39] . Interestingly, in the bone marrow where HEp3 DTCs do not proliferate, the NR2F1 knockdown caused a reduction in BM DTC burden ( Fig. 7e ). This may be due to NR2F1-induced survival because knockdown of this TF in the BM-HEp3 cells that express higher NR2F1 mRNA levels than the proliferative counterparts, also resulted in less dormant tumour cells recovered in vivo ( Supplementary Fig. 6f,g ). We next tested the function of NANOG, which is downregulated upon NR2F1 depletion in BM-HEp3 cells ( Supplementary Fig. 6f ). To our surprise, unlike NR2F1 knockdown, NANOG knockdown reactivated dormant BM-HEp3 cells in vivo ( Supplementary Fig. 6h ). It is possible that NR2F1-induced NANOG in BM-HEp3 regulates quiescence—and that NR2F1 regulates directly target genes involved in survival. Thus, depending on the organ microenvironment, NR2F1 might fulfil quiescence and/or survival functions and the former may be executed by NANOG in the BM. Finally, we tested the link between atRA, NR2F1 and TGFβ2 signalling because we found that in the bone marrow TGFβ2 induces dormancy [6] and this cytokine mRNA was upregulated in PCa DTCs from NED versus ADV patients. In addition, atRA is abundant in the BM where it regulates HSC self-renewal and differentiation [40] , [41] . Treatment of T-HEp3 cells with atRA induced TGFβ2 mRNA, but this was not mediated by NR2F1 ( Supplementary Fig. 6i ). These data support a model where microenvironmental signals propagated by RA and TGFβ2 signalling might cooperate to induce quiescence and survival of DTCs in the bone marrow. The role of NR2F1 in quiescence induction and cell lineage commitment [42] might explain why it is downregulated in proliferative tumours and how its re-expression by specific microenvironments or by ‘epigenetic therapies’ induces stable dormancy in aggressive tumour cells ( Fig. 8 ). Our findings, while limited to some extent by the use of human cancer cell lines and mouse models, still appear to provide relevant information regarding human DTC dormancy. For example, NR2F1 and TGFβ2 are more frequently upregulated in DTCs from NED than ADV PCa patients. This strongly argues that NR2F1- and TGFβ2-driven dormancy programmes may be extremely long-lived in DTCs in human bone marrow ( Fig. 8 ). Further, these prostate cancer DTCs had a significant upregulation of the whole dormancy signature identified in our dormancy model, further arguing that there may be a commonality in the mechanisms that reprogramme tumour cells into dormancy. This is also supported by our findings that the same signature predicts for longer metastasis-free periods in breast cancer patients with ER+ luminal tumours [7] . In our system of BM DTC dormancy NR2F1 drives growth arrest via SOX9, RARβ and NANOG, while NR2F1 itself favours survival. In D-HEp3 cells NR2F1 drives quiescence. How these different functions are coordinated is still unknown but it may be related to how these cells are reprogrammed into dormancy [3] , [6] . 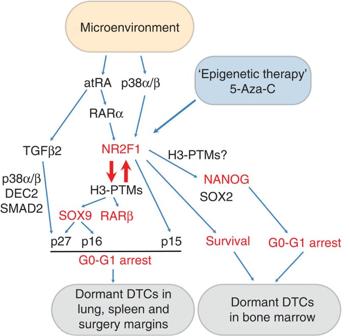Figure 8: Integrative scheme of NR2F1 functions and the regulation of DTC fate. DTCs that arrive to specific microenvironments (for example, lung and bone marrow) might integrate stress signals imposed by dissemination (p38α/β activation), by the new microenvironment and growth-restrictive signals that maintain normal organ function (atRA+p38α/β activation). These signals jointly result in NR2F1 upregulation, which can in turn induce a quiescence programme via the induction of CDK inhibitors (that is, p16). This is executed by another set of TFs that include at least SOX9 and RARβ. In lung, spleen and surgery margins, the NR2F1-regulated quiescence programme seems to be important to maintain dormancy, while in the bone marrow NR2F1 appeared to primarily regulate survival of DTCs. NR2F1 was also found to regulate the expression of the two key pluripotency genes,NANOGandSOX2. A division of labour between NANOG and NR2F1 occurs in BM DTCs where growth arrest signals are regulated by NANOG, while survival pathways are subjected to NRF21 functions. The ability of NR2F1 to coordinate these programmes long term may be because of its ability to generate global changes in histone-H3-PTMs. atRA also regulates the induction of TGFβ2 in malignant cells that further induces signals in the dormancy programme by inducing DEC2 via canonical and noncanonical TGFβ2 signalling; this is independent of NR2F1. Finally, the dormancy programme may be manipulated to favour dormancy maintenance using 5-Aza-C combined with atRA as an epigenetic therapy. This reprogramming protocol may also be used to study how dormant cells survive in quiescence and design antisurvival therapies that target quiescent DTCs. Figure 8: Integrative scheme of NR2F1 functions and the regulation of DTC fate. DTCs that arrive to specific microenvironments (for example, lung and bone marrow) might integrate stress signals imposed by dissemination (p38α/β activation), by the new microenvironment and growth-restrictive signals that maintain normal organ function (atRA+p38α/β activation). These signals jointly result in NR2F1 upregulation, which can in turn induce a quiescence programme via the induction of CDK inhibitors (that is, p16). This is executed by another set of TFs that include at least SOX9 and RARβ. In lung, spleen and surgery margins, the NR2F1-regulated quiescence programme seems to be important to maintain dormancy, while in the bone marrow NR2F1 appeared to primarily regulate survival of DTCs. NR2F1 was also found to regulate the expression of the two key pluripotency genes, NANOG and SOX2 . A division of labour between NANOG and NR2F1 occurs in BM DTCs where growth arrest signals are regulated by NANOG, while survival pathways are subjected to NRF21 functions. The ability of NR2F1 to coordinate these programmes long term may be because of its ability to generate global changes in histone-H3-PTMs. atRA also regulates the induction of TGFβ2 in malignant cells that further induces signals in the dormancy programme by inducing DEC2 via canonical and noncanonical TGFβ2 signalling; this is independent of NR2F1. Finally, the dormancy programme may be manipulated to favour dormancy maintenance using 5-Aza-C combined with atRA as an epigenetic therapy. This reprogramming protocol may also be used to study how dormant cells survive in quiescence and design antisurvival therapies that target quiescent DTCs. Full size image The plasticity in NR2F1 expression suggests that specific signals might restore NR2F1 high levels in disseminated disease as observed in DTCs from PCa patients who had NED from 7 to 18 years. In agreement with these findings, NR2F1 expression was higher in prostate cancer patient’s tumours after hormonal therapy [18] . Thus, microenvironmental signals or therapy may induce NR2F1 re-expression and determine the rate at which residual disease reactivates. A potential utility might be the detection of NR2F1, SOX9, RARβ and possibly NANOG in DTCs as biomarkers. These may pinpoint DTCs in a dormant state and with latent capacity to reactivate or that responded to epigenetic therapies [43] . These could also be tested in CTCs in M0 patients to identify precursors of dormant DTCs or re-circulating dormant tumour cells. Alternatively, as with DTCs, testing these markers on CTCs may be informative on response to therapies that activate the dormancy mechanisms. Our data reveal something particular about NR2F1 in that in malignant cells that entered dormancy it coordinates quiescence, survival and the expression of pluripotency genes ( Fig. 8 ). In this dormancy context, NANOG may help to maintain the quiescence phase induced by NR2F1 upregulation. We cannot rule out that the pluripotency genes may allow DTCs to survive and avoid differentiation, senescence or at some point reactivate. The stability and also plasticity of the dormant phenotype were linked to the ability of NR2F1 to induce global repressive chromatin states as evidenced by enrichment in H3K27me3 and H3K9me3 marks upon spontaneous or Aza+atRA-induced reprogramming ( Fig. 8 ). While globally NR2F1 induces a chromatin-repressive state, the regulation by NR2F1 of H3K4me3 marks in its own and SOX9 and RARβ promoters indicate that it can also regulate local active chromatin changes. Specific microenvironments may contain cues (for example, RA and TGFβ2) that in malignant tumour cells receptive to these signals may activate a dormancy programme. Remarkably, NR2F1 appears to execute such a programme in occult DTCs in several organs and in the surgery margins by inducing a specific combination of pluripotency (NR2F1 high /[NANOG/Sox2] high ) and quiescence (SOX9 high /RARβ high /p27 high ) genes. This may explain the longer metastasis-free periods in patients carrying NR2F1 high tumours (and putative NR2F1 high DTCs) [7] , [18] . Our results show that ‘epigenetic therapies’ (demethylating agents) currently used in patients [43] could induce dormancy when used at low doses and combined with atRA ( Fig. 8 ). Remarkably, the key genes (for example, RARβ and CDKN1A) that were induced by the p38α/β [3] , [7] were also induced by demethylating agents [43] . Our combination of ‘differentiation’ and ‘epigenetic’ therapies or the combination of specific transcription factors (for example, NR2F1, SOX9 and RARβ) might be a strategy to generate induced dormant cancer cells. This may provide the basis for designing new therapeutics to prevent residual disease from reactivating after tumour surgery and/or chemotherapy. Such ‘dormancy-inducing therapies’ could be used to convert residual proliferative tumour cells into dormancy and/or prevent pre-existing dormant cells from re-awakening. On the other hand, in vitro generation of induced dormant cancer cells or dormant DTCs obtained from different microenvironments may allow discovering the survival mechanisms that allow them to persist over time and eradicate them. BM DTCs may require NR2F1 for survival, suggesting that targeting the downstream executors of the survival programme, may be useful to eliminate DTCs in cancers that primarily target bone such as prostate cancer and ER+ luminal breast cancer. This also implies that a global single approach to target all disseminated cells found in different tissues in a patient may not be the best scenario. Perhaps a combination of drugs that specifically target the key dormancy-regulating genes in specific microenvironments might be needed. Cell lines Tumorigenic (T-HEp3) HEp3 cells were derived from a lymph node metastasis from a HNSCC patient as described previously [26] and kept as patient-derived xenografts in CAMs. Dormant D-HEp3 cells were obtained by passing T-HEp3 cells for more than 40 generations in vitro [26] . Dormant (BM-HEp3) and proliferative (Lu-HEp3) cells derived from bone marrow- and lung-derived T-HEp3 DTCs were described previously [6] . When cultured in vitro all these cells were passaged in DMEM cell growth medium (Dulbeco’s modified medium with 10% of fetal bovine serum (FBS) and 100 U penicillin/0.1 mg ml −1 streptomycin). The 4T1 cells are derived from a single spontaneous primary mammary tumour that arose in a wild-type BALB/c mouse [44] . ShNR2F1miR cells were generated by TURBO-RFP-shNR2F1miR encoding lentivirus infection of T-HEp3 cells then selected with puromycin (2.5 μg ml −1 ). For the MMTV-myc studies, primary cultures from MMTV-myc mouse tumours [45] were transfected with pGS5-empty or pGS5-Nr2f1. Briefly, MMTV-myc tumour cells were isolated by adding collagenase for 30 min at 37 °C. Then, suspension of cells were plated in 10 cm dishes to allow for fibrosblast to attach and the resuspended cells were treated with PBS-EDTA (2 mM) for 15 min at 37 °C to reach single-cell suspension. Finally, tumour cells were plated and grown in DMEM:F12 medium with 5% horse serum, EGF (20 ng ml −1 ), Hydrocortisone (0.5 mg ml −1 ), cholera toxin (100 ng ml −1 ), insulin (10 μg ml −1 ), penicillin/streptomycin (1 × solution). pCDNA3.1(+) was used as a selection marker by co-transfection in a ratio 10:1. G418-resistant cells were selected by cloning dilution. SQ20b, MCF-7 and FaDu cells were obtained from ATCC and were grown in the same medium as T-HEp3 cells. 4T1 and PC3 were obtained from ATCC and grown in RPMI medium with 10% of FBS. Reprogramming protocol After seeding, T-HEp3 cells were grown in DMEM high-glucose media plus 10% of charcolized serum and penicillin/streptomycin and the addition of Azacytidyne (5-AzaCytidine, 5 nM) for 24 h. Next day, fresh AzaC (5 nM) was added (See Supplementary Fig. 4f ). Then, media was changed for serum-free media plus atRA (2 μM) for 48 h. All these treatments are designed as pre-reprogramming step (pre-step). Subsequently, the media was changed for normal growing media without the addition of any drug (post-step) and with this started the post-reprogramming protocol. Reagents and antibodies Charcoal Stripped FBS One Shot (Gibco, Life technology, NY, USA), 5-azadeoxycytidine (Sigma, MO, USA), atRA (Sigma), senescence beta galactosidase kit (Cell Signaling, MA, USA), Dual luciferase reporter system (Promega, Wisconsin, USA), trizol (Invitrogen, NY, USA), NR2F1 antibody for western blot (R&D systems, MN, USA), NR2F1 antibody for IF and IHC (Abcam, MA, USA), p27, p21 and cleaved-caspase 3 (Cell signaling), Ki67 (Invitrogen) and SOX9 (Millipore, MA, USA). Human NR2F1 plasmid was a kind gift from Dr Gilles Salbert (Rennes University, France). Mouse NR2F1 plasmid was a kind gift from Dr Lorraine Gudas (Weill Cornell Medical College). All primary antibodies for IF/IHC were used at a dilution of 1:100. Xenograft studies All animal studies were approved by Institutional Animal Care and Use Committees (IACUC) at the Mount Sinai School of Medicine Protocol ID: 08–0366. Tumour growth on chick embryo CAMs or Balb/c nude mice has been described previously [46] . Briefly, 150 × 10 3 T-HEp3 cells were inoculated on the chicken embryo chorioallantoic membrane and allowed them to grow for the indicated times in each experiment (from 4 to 7 days). Dormant D-HEp3 and BM-HEp3 cells were inoculated into CAMs at 500 × 10 3 cells per egg. For atRA in vivo experiments, 150 × 10 3 T-HEp3 cells were resuspended in 50 μl PBS in the presence of atRA (2 μM) or DMSO and inoculated into each CAM. Twenty-four hours post inoculation 50 μl of PBS plus atRA (2 μM) or DMSO were added on top of each egg. On day 4, the same treatment was repeated. Tumours were harvested on day 5, minced, digested with collagenase-1A (Sigma—C9891) for 30 min at 37 °C and tumour cells, recognized by their very large diameter, were counted with a hemocytometer. For serial transplantation studies of HEp3 tumours on CAM, HEp3 tumours were minced and dissociated with collagenase-IA, tumour cells were counted and a single-cell suspension (150 × 10 3 cells in 50 μl PBS) from each tumour was reinoculated on CAMs. For RNA interference studies, transfections of cells with siRNAs targeting the desired sequences or control scrambled siRNA were performed as previously described [3] . Twenty-four hours after transfection 150 × 10 3 cells were inoculated on the CAM of 9–10-day-old chicken embryos (Charles River). Four days post inoculation, the number of tumour cells per nodule was counted. siRNAs knockdown were analysed with QPCR. For the HEp3 xenograft studies, 750 × 10 3 cells were injected subcutaneously in 8-week-old female BALB/c nu/nu mice (Jackson Laboratories) in the interscapular region. Mice were inspected every 48 h and arising tumours were measured with calipers in two perpendicular diameters. Mice were kept (~14 days) until primary tumours developed and grew up to ~500–800 mm 3 . Mice were then injected with anaesthetics ketamine 80–120 mg i.p. and xylazine 5 mg i.p, and an incision of ~1 cm above the base of the tumour was performed. This allows gently scoop-out the tumour tissue and leaving sufficient skin to close the wound with sutures. Sutures were performed using a wound clipper. In the DOX-induced depletion of NR2F1 studies, mice were injected i.p. with 25 mg kg −g of DOX or vehicle every 48 h. For the MMTV-myc tumour studies, 1,000 or 10,000 MMTV-Myc-vector or MMTV-Myc-NR2F1 cells were orthotopically injected in the mammary fat pad of synergetic FvB mice. Tumours were detectable from day 7 and were measured every other day. Animals were killed when tumours reached 500 mm 3 size. IHC and IF assays Paraffin-embedded sections from human HNSCC tumours and lymph node metastasis and breast carcinoma tissues were stained for NR2F1 expression after quenching endogenous peroxidase activity. Binding of the primary antibody was carried out at 4 °C overnight, detected by anti-rabbit secondary antibody (1 h at room temperature) and revealed using DAB Chromagen. Paraffin-embedded sections from T-HEp3 and D-HEp3 tumours were stained for the followed antigens: SOX9 (dilution of Ab 1:150 for D-HEp3 and 1:75 for T-HEp3), NR2F1 (1:100 for D-HEp3 and 1:50 for T-HEp3) and Ki67 (dilution of ab 1:100). For immunofluorescence assays, tumour cells seeded in coverslips were fixed with 4% paraformaldehyde (PFA) in PBS and were permeabilized with 0.1% Triton X-100. Cells were then blocked with PBS containing 3% normal goat serum. Gene expression profiling from T- and D-HEp3 cells in vivo GFP-tagged T-HEp3 and D-HEp3 cells were inoculated and allowed to grow (T-HEp3) or enter dormancy (D-HEp3) for 1 week. Then 5 T-HEp3 tumours or 5 D-HEp3 dormant nodules were processed for FACS and GFP+ cells were used to extract RNA. This RNA (10 μg) was used to perform gene expression profiling using the Affymetrix HG-U133-PLUS2 arrays. The analysis of the gene expression profiles was performed as described in ref. 3 and the data are deposited in the Gene Expression Omnibus (GEO) under the accession number GSE58588. Additional methods can be found to be associated with the profiles in the GEO database. The following link has been created to allow review of record GSE58588 while it remains in private status: http://www.ncbi.nlm.nih.gov/geo/query/acc.cgi?token=ovilmukmxluvpaj&acc=GSE58588 Human prostate cancer DTC isolation and expression profiling Individual prostate cancer DTCs were isolated from the bone marrow of post-radical prostatectomy patients with NED (dormant disease) or ADV [31] . Samples were obtained from patients who signed written informed consent. The study was approved by the Cancer Consortium institutional review board at the Fred Hutchinson Cancer Research Center and the University of Washington (Protocol no. 7350). NED patients showed undetectable PSA level (<0.1 ng ml −g ) 7–18 years after prostatectomy. ADV patients showed disease progression with failed treatment or existing distant metastasis. Seven individual NED cells (four patients) and 37 ADV cells (six patients) were amplified using the WT-OviationTM one-direct system (NuGEN) and single-cell gene expression was analysed by Agilent 4 × 44 K Human Microarrays. The analysis of the gene expression profiles of single cells obtained from patients with advanced disease and patients with no evidence of disease was performed on the profiles in GEO database under the accession number GSE48995. All isolation methods and procedures are described therein. The following link has been created to allow review of record GSE48995 while it remains in private status: http://www.ncbi.nlm.nih.gov/geo/query/acc.cgi?token=ndclzsckieyygte&acc=GSE48995 . Senescence assays Tumours were harvested, digested with collagenase-1A (Sigma—C9891) for 30 min at 37 °C and then the manufacturer’s protocol for senescence detection (Cell Signaling, no. 9860S) was followed. RNA interference Transfections of siRNAs targeting the desired sequences or scrambled siRNA were performed using siPORT NeoFX (Ambion). Detached cells were resuspended and overlaid on the transfection complexes. After 24 h under normal cell culture conditions, cells were either used for in vivo experiments or lysed for immunoblotting and/or qPCR. Human siNR2F1 sequence sense: 5′-CUCUCAUCCGCGAUAUGUU-3′; antisense: 5′-AACAUAUCGCGGAUGAGAG-3′ (SIGMA, SASI_Hs01_00095428/AS). Human siNANOG sequence sense: 5′-GUGUGUACUCAAUGAUAGA-3′, antisense: 5′-UCUAUCAUUGAGUACACAC-3′ (SIGMA, SASI_Hs01_00163355/AS). Human siSOX9 sequence sense: 5′-CGUGUGAUCAGUGUGCUAA-3′; antisense: 5′-UUAGCACACUGAUCACACG-3′ (SIGMA, SASI_Hs01_00240733/AS). Human siRARβ sequence sense: 5′-CAUUGCUGGAAGCACUAAA-3′; antisense: 5′-UUUAGUGCUUCCAGCAAUG-3′ (SIGMA, SASI_Hs01_00237846/AS). Immunoblotting, RT–PCR and qPCR Images for immunoblotting have been cropped for presentation. Full-size images are presented in Supplementary Figs 7–11 . RT–PCR and qPCR were performed as described previously [3] . NR2F1 human forward primer: 5′-GCCTCAAAGCCATCGTGCTG-3′, NR2F1 human reverse primer: 5′-CCTCACGTACTCCTCCAGTG-3′, SOX9 human forward primer: 5′-CACTCCTCCTCCGGCATG-3′, SOX9 human reverse primer: 5′-GGCTGCACGTCGGTTTTGG-3′, RARβ human forward primer: 5′-GTACCACTATGGGGTCAGCG-3′, RARβ human reverse primer: 5′-CGACAGTATTGGCATCGATTCC-3′, NANOG human forward primer: 5′-CTAAGAGGTGGCAGAAAAACA-3′, NANOG human reverse primer: 5′-CTGGTGGTAGGAAGAGTAAAGG-3′, SOX2 human forward primer: 5′-GTTGTCAAGGCAGAGAAGAG-3′, SOX2 human reverse primer: 5′-GAGAGAGGCAAACTGGAATC-3′, TUBULIN human forward primer: 5′-CCCTCCAAGCTCTACTCT-3′, TUBULIN human reverse primer: 5′-GACCAAGGCTGGTCTCTTTC-3′, HES-1 human forward primer: 5′-CCCAGCCAGTGTCAACACGACA-3′, HES-1 human reverse primer: 5′-GGTACCGCCCTTACCTTTCTGTGC-3′, p27 human forward primer: 5′-GGTTAGCGGAGCAATGCGCA-3′, p27 human reverse primer: 5′-AACCGGCATTTGGGGAACCGTC-3′, p15 human forward primer: 5′-TGGGGTGGGAAAGTGGATTGCA-3′, p15 human reverse primer: 5′-CCCAGTGCAGAGGTGTTCAGGTCT-3′, p16 human forward primer: 5′-GCTGCTCACCTCTGGTGCCAAA-3′ and p16 human reverse primer: 5′-ACCTGCGCACCATGTTCTCG-3′. Detection of DTCs via Alu -qPCR Human cells within mouse BM, lungs and spleen were detected by real-time Alu -qPCR, essentially as described [47] . Briefly, BM flushes were snap-frozen in liquid nitrogen and the genomic DNA was extracted using the Extract-N-Amp kit from Sigma (XNAT2-1KT). Genomic DNA (30 ng) was used per PCR reaction. Amplification of mice GAPDH was used as an internal control for the total amount of tissue. The ratio between hAlu and mGAPDH is used for comparative purposes between experimental groups. The primers for hAlu sequences and mice GAPDH were: hAlu sense (5′-ACGCCTGTAATCCCAGCACTT-3′) and hAlu antisense (5′-TCGCCCAGGCTGGGTGCA-3′), mGAPDH FW (5′-ATGGTGAAGGTCGGTGTGA-3′) and mGAPDH RV (5′-CGTTGATGGCAACAATCTC-3′). Each assay included two negative controls (water and genomic DNA extracted from BM, lung and spleen from a mouse that has not been injected with human cells), a positive control (human genomic DNA) and the experimental samples in triplicate. The actual number of tumour cells present in each tissue sample was determined using a standard curve generated by serial dilution of HEp3 cells. Briefly, organ-specific cells were collected from nude mice that did not bear tumours. HEp3 cells were serially diluted into mice organ-specific single-cell suspensions and the genomic DNA was extracted and amplified. The actual number of tumour cells could be determined over a range of 10–1,000 cells per BM, 100–10,000 cells per spleen and over 100–1,000,000 cells per lung. Sphere-forming assay After the pre-reprogramming protocol, T-HEp3 cells were seeded in low-attachment six-multi-well plates (100 × 10 3 cells per well) in stem cell media (DMEM:F12, B27 supplement, EGF). Sphere formation was observed by light microscope and spheres were counted on day 6. MMTV-myc cells: MMTV-myc control cells or MMTV-myc-Nr2f1 cells were trypsinized, dissociated by pipetting and filtering through a 40-μm pore cell strainer. In all, 1 × 10 5 cells per condition were plated by triplicates in ultralow adhesion six-well plates (Corning, Corning, NY, USA) and incubated in serum-free F12/DMEM 50:50 medium (Cellgro, Mediatech Inc, Manassas, VA, USA) supplemented with 20 ng ml −l EGF and 1:50 B27 Supplement (Invitrogen, Carlsbad, CA, USA). Flow cytometry For the characterization of the progenitor containing compartments, each well was dissociated with PBS-EDTA at 37 °C with gentle shaking, filtered through a 40-μm cell strainer and incubated with PE or APC-conjugated anti-CD24 Ab (BD Pharmingen, San Jose, CA, USA), APC-conjugated anti-CD29 Ab (Invitrogen, Camarillo, CA, USA). Sequenom array The bisulfite PCR primers for the Sequenom array were designed using the EpiTYPER software ( Supplementary Table III ). Genomic DNA from each sample was prepared using the QIAamp DNA mini kit (Qiagen) and the concentration and quality were determined by measuring the absorbance at 260 and 280 nm in a spectrophotometer (NanoDrop 8000, Thermo Scientific). DNA was subjected to bisulfite modification by using the EZ DNA Methylation kit (Zymo Research). Purified DNA samples were forwarded to Sequenom MassARRAY core facility at the Cornell University Institute of Biothechnology. ChIP ChIP was performed as previously described and followed by qPCR analysis [48] . The antibodies used for the immunoprecipitation were the following: H3K4me3 (ab1012, Abcam), H3K9me3 (ab8898, Abcam) and H3K27ac (ab4729, Abcam). Real-time PCR reactions (Roche) were performed in triplicates using primers for the correspondent genomic regions. Fold enrichment over 1% input was calculated using the 2DeltaCt method. Primers for ChiP are described in Supplementary Table IV . Statistical analysis For DTC detection experiments, the P values were estimated using Mann–Whitney nonparametric test with one-tailed P values≤0.05 considered significant. For all the rest of the experiments unpaired t -test were used with a 95% confidence. For in vitro experiments, a minimum of triplicates per group and repetition of at least three times was applied to achieve reproducibility. For in vivo experiments a minimum of five tumours for CAM assays and a minimum of eight mice was assessed to achieve reproducibility. Accession codes . Gene Expression Omnibus under the accession number GSE58588 and GSE48995 . How to cite this article: Sosa, M. S. et al. NR2F1 controls tumour cell dormancy via SOX9- and RARβ-driven quiescence programmes. Nat. Commun. 6:6170 doi: 10.1038/ncomms7170 (2015).